Monolithically integrated mid-infrared lab-on-a-chip using plasmonics and quantum cascade structures The increasing demand of rapid sensing and diagnosis in remote areas requires the development of compact and cost-effective mid-infrared sensing devices. So far, all miniaturization concepts have been demonstrated with discrete optical components. Here we present a monolithically integrated sensor based on mid-infrared absorption spectroscopy. A bi-functional quantum cascade laser/detector is used, where, by changing the applied bias, the device switches between laser and detector operation. The interaction with chemicals in a liquid is resolved via a dielectric-loaded surface plasmon polariton waveguide. The thin dielectric layer enhances the confinement and enables efficient end-fire coupling from and to the laser and detector. The unamplified detector signal shows a slope of 1.8–7 μV per p.p.m., which demonstrates the capability to reach p.p.m. accuracy over a wide range of concentrations (0–60%). Without any hybrid integration or subwavelength patterning, our approach allows a straightforward and cost-saving fabrication. Mid-infrared spectroscopy is one of the main techniques for chemical sensing. Molecules can be identified through their unique pattern of absorption lines, which give rise to the ‘fingerprint region’ for mid-infrared wavelengths. This operational principle is successfully used in a number of applications including chemical sensing, environmental monitoring, as well as medical and microbiological diagnosis. A mid-infrared spectrometer typically consists of a broadband thermal emitter and broadband detector, external optics, as well as a Fourier-transform infrared spectrometer (FTIR). Depending on the actual application, these discrete building blocks must be aligned with a multi-pass gas cell or a fluidic cell, holding the analyte. A challenging task is to make mid-infrared spectroscopy accessible to remote areas, where conventional power supply and laboratory equipment is not available or possible [1] . The steadily increasing demand for more compact and cost-effective sensing solutions requires monolithic integration to replace table-top systems with portable devices that incorporate all necessary optical components and functionality onto a single chip. A key issue of miniaturization is the waveguide that should provide a strong interaction with the environment while still guiding the light with high efficiency. An elegant solution is the surface plasmon polariton (SPP) waveguide in which the electromagnetic wave propagates along a metal/dielectric interface with an evanescent decay on both sides [2] . In the visible and near-infrared spectral range, the ability of metallic micro- and nanostructures to confine and locally enhance light on the subwavelength scale is an enormous benefit for many applications [3] . The resonant interaction between photons and free-electron plasmas has already solved a number of fundamental problems in sensing [4] , [5] , imaging [6] and on-chip communication [7] . In the mid-infrared, plasmonics are an often overlooked field. Owing to the different material response, the knowledge from shorter wavelengths cannot be easily transferred to the mid-infrared [8] , [9] . At visible and near-infrared wavelengths, noble metals have a negative permittivity with an absolute value comparable to that of typical dielectrics, thereby enabling deep subwavelength confinement. In contrast, the negative permittivity in the mid-infrared is much larger, leading to the fact that surface waves are weakly bound to the metal-dielectric interface with an evanescent decay penetrating deep into the dielectric medium. The weak confinement is a main issue, as to why mid-infrared plasmonics have not been as broadly adopted. Despite these challenges, mid-infrared plasmonics have been demonstrated for a few very promising applications, such as beam-shaping [10] , sensing [11] and nano-focusing [12] . Here we demonstrate a monolithically integrated lab-on-a-chip based on mid-infrared absorption spectroscopy by solving two major issues that previously inhibited the integration and downscaling of the laser, waveguide and detector. First, an epitaxial structure that can serve as a coherent light source and as a detector allows a compact yet fully functional sensing device. Second, the interaction between the electromagnetic wave and the analyte is managed through an SPP waveguide. This waveguide offers both a high coupling efficiency of 30–50% as well as a strong interaction with the environment. With the entire device submerged in a mixture of ethanol in water, we achieve a resolution of 0.06% over a large dynamic range of concentrations from 0 to 60%. Concept The on-chip sensor comprises a laser, an SPP waveguide and a detector, monolithically integrated onto the same substrate. 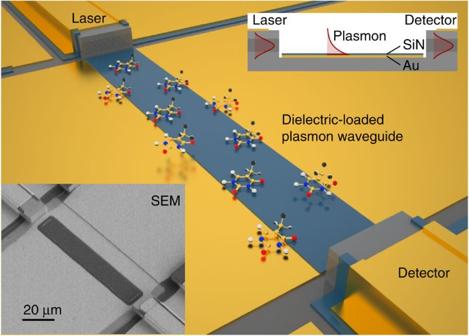Figure 1: Monolithic mid-infrared on-chip sensor. The device comprised of a laser, a SPP waveguide and a detector, monolithically integrated on the same substrate. The upper inset shows the cross section of the structure and the lower inset the corresponding scanning electron microscope (SEM) image of the fabricated device. Figure 1 shows a sketch and an scanning electron microscope image of the fabricated device and its use as a chemical sensor. The light emitted from the laser is coupled to a surface wave that propagates via the plasmon waveguide to the detector. This SPP waveguide acts as an interaction zone for chemical substances. Compared with dielectric waveguides, the major part, 96%, of the mode stays outside in the fluid, providing a strong interaction. By applying a thin dielectric layer on top of an unpatterned gold surface, the mid-infrared SPP is compressed by an order of magnitude. In parallel, the dielectric is used for lateral confinement to reduce the waveguide losses in the narrow waveguide. The enhanced confinement because of the thin dielectric layer allows the direct excitation and detection of SPPs with a ridge laser and detector. For this, we use a bi-functional quantum cascade laser/detector (QCLD) active region [13] . The capability of both generating and detecting mid-infrared light with the same epilayer structure, simply by changing the applied bias, makes this bi-functional structure an ideal candidate for monolithic devices [14] . We have significantly improved the performance of the active region by further optimization to prevent thermal back-filling. At room temperature, our fabricated devices have a pulsed output power of up to 200 mW for the laser and a responsivity of 46 mAW −1 for the on-chip detector at the laser wavelength. This responsivity is one order of magnitude higher than reported for discrete quantum cascade detectors (QCDs) at room temperature [15] , [16] . In order to fulfil the polarization selection rule of intersubband transitions, electric field perpendicular to the surface, discrete QCDs require special techniques. This can be achieved with a 45° incident angle by rotating normal incident light with gratings or more sophisticated photonic crystals cavities [17] . For an on-chip detector, light can be directly coupled from a waveguide to the detector, improving the overall performance of the device significantly. This allows the use of a ridge detector with a higher absorption efficiency (higher responsivity) and a smaller electrical area (lower noise). Figure 1: Monolithic mid-infrared on-chip sensor. The device comprised of a laser, a SPP waveguide and a detector, monolithically integrated on the same substrate. The upper inset shows the cross section of the structure and the lower inset the corresponding scanning electron microscope (SEM) image of the fabricated device. Full size image With the bi-functional QCLD and the dielectric-loaded SPP (DLSPP) waveguide, we combine two technologies that are ideally suited for on-chip sensing applications and are fully compatible with each other. Both give rise to the same polarization (electric field perpendicular to the surface) and can be fabricated onto the same substrate without any hybrid integration approaches. Thus, the presented on-chip sensor can be fabricated for basically the same cost as the mid-infrared laser (QCL) alone. Increasing the confinement of mid-infrared SPPs In the mid-infrared, SPPs propagating on a metal–air interface are weakly confined and penetrate deeply into the dielectric material. Pendry et al. [18] proposed patterning the metal surface with resonant grooves to modify the propagation properties in such a way that electromagnetic waves are strongly bound to the interface. These so-called spoof or designer SPPs are collective excitations of optical modes in the grooves with subwavelength periodicity resulting in an effective media with a plasma-like response. Our approach is different. We apply a thin dielectric stripe on top of an unpatterned metal surface, which provides propagation properties similar to spoof plasmons, but without the need for subwavelength patterning. This dielectric layer produces an increase of the effective modal index, enabling the propagation of well-confined mid-infrared plasmon waves. Depending on the thickness of the dielectric layer, in our case SiN x , the evanescent decay length into the air can be adjusted over a broad range, 2–50 μm ( Fig. 2a ). A SiN x layer, a few hundred nanometres thick, is sufficient to squeeze the mode by one order of magnitude. 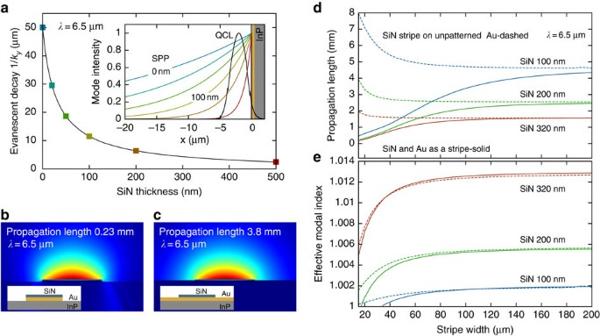Figure 2: Simulations of DLSPP waveguides. (a) Vertical confinement due to dielectric loading. A thicker dielectric layer leads to a better confinement of the SPP. The inset shows the modal intensity profile of the SPP for different SiNxthickness, corresponding to the points at 0, 20, 50, 100, 200 and 500 nm, as well as the mode of the QCL/QCD ridge waveguide. (b) Simulated 2d mode profile of the DLSPP waveguide with a 200-nm-thick and 15-μm wide SiNxstripe on top of a gold stripe, and (c) on an unpatterned gold surface. (d) Influence of the stripe width and the SiNxlayer thickness on the propagation length and (e) the effective modal index for the two waveguide configurations (gold stripe as solid lines and gold surface as dashed lines). For narrow waveguides, the additional loss because of the metal edges leads to a marked reduction of the propagation length. In this case, dielectric loading can improve not only the confinement, but also the propagation length significantly. Figure 2: Simulations of DLSPP waveguides. ( a ) Vertical confinement due to dielectric loading. A thicker dielectric layer leads to a better confinement of the SPP. The inset shows the modal intensity profile of the SPP for different SiN x thickness, corresponding to the points at 0, 20, 50, 100, 200 and 500 nm, as well as the mode of the QCL/QCD ridge waveguide. ( b ) Simulated 2d mode profile of the DLSPP waveguide with a 200-nm-thick and 15-μm wide SiN x stripe on top of a gold stripe, and ( c ) on an unpatterned gold surface. ( d ) Influence of the stripe width and the SiN x layer thickness on the propagation length and ( e ) the effective modal index for the two waveguide configurations (gold stripe as solid lines and gold surface as dashed lines). For narrow waveguides, the additional loss because of the metal edges leads to a marked reduction of the propagation length. In this case, dielectric loading can improve not only the confinement, but also the propagation length significantly. Full size image The so-called DLSPPs have already been investigated both theoretically and experimentally for telecommunication wavelengths [19] , [20] . There, the increased vertical confinement has a minor role as the SPPs are already well confined. The main advantage is the increased propagation length for SPPs with high lateral confinement. In the mid-infrared, dielectric loading solves both issues. It enables the propagation of surface plasmons that are strongly bound to the interface and it significantly increases the propagation length for narrow waveguides. Although loss within the dielectric layer can be neglected by choosing the right material, increased vertical confinement always goes with an increase in ohmic loss owing to the higher field intensity at the metal interface. For high lateral confinement with narrow metal stripes, the waveguide loss is dominated by scattering on the metal edges ( Fig. 2b ). The obvious solution is to eliminate these metal edges, which is possible with dielectric loading. To achieve this, the dielectric layer is patterned as a stripe on top of an unpatterned gold surface ( Fig. 2c ). For a 15-μm-wide plasmonic waveguide, the dielectric guiding yields an increased propagation length of one order of magnitude while providing the same lateral and enhanced vertical confinement. For the fabricated structures (15 μm wide with 200 nm SiN x ), our simulations show a propagation length of 2–4 mm, depending on the material parameters [21] , [22] . Tetienne et al. [23] obtained a propagation length of 1.8 mm for the 60-μm-wide gold stripe at λ =7.5 μm from their experiments, which is one order of magnitude lower than the theoretic value of SPP propagating on an air/gold interface. This can be attributed to scattering on the metal edges and partly to fabrication imperfections, for example, surface roughness. Dielectric loading helps both to eliminate the metal edges and to reduce roughness scattering with an increased effective modal index. Figure 2d depicts the influence of the stripe width on the propagation length, and Fig. 2e depicts the modal index for both waveguide configurations (gold stripe as solid lines and SiN stripe atop gold surface as dashed lines). When gold is used for lateral confinement, the propagation length markedly reduces with decreasing waveguide width. The situation changes when the dielectric layer is used to laterally confine the SPP. There, a decreased waveguide width leads to a slight increase of the propagation length. Exciting and detecting SPPs with a bi-functional QCLD The most common techniques to couple light from free space to an SPPs are based on prism or grating coupling [2] . An alternative way to excite guided modes is spatial mode matching, commonly referred to as end-fire coupling. This can be achieved either by precisely focusing light onto the end of the waveguide or, as in our case, by placing the waveguide in the direct vicinity of the laser. As intersubband transitions interact with the same polarized light as supported by SPP waveguides, an SPP mode can be directly excited with a QCL [23] . 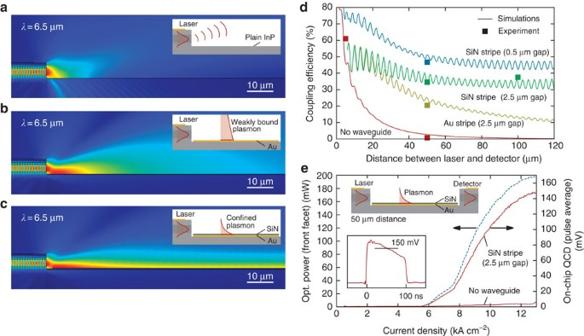Figure 3: Excitation and detection of SPPs. (a) Without waveguide light couples to free space and partially into the substrate. (b) An SPP can be excited on the gold surface, but is weakly bound to the interface. (c) The 200-nm-thick SiNxlayer on top of the gold surface leads to an increased confinement. Owing to the high confinement, this SPP can be coupled directly to a detector. (d) Coupling efficiency from the laser to detector facet over the distance between them, with the simulation as curves and the experiment as points. (e) Detector signal into 50 Ω compared with the laser power (front facet) over the laser current density for a distance of 50 μm. The inset shows the time-resolved detector signal. Opt., optical. Figure 3a shows the finite element simulation result of the emission from an etched laser facet without a waveguide. Laser light is emitted mainly to free space and partly into the substrate. By adding a gold layer in the direct vicinity of the laser facet, a surface plasmon can be excited. As this SPP is weakly confined (50 μm), it cannot be coupled efficiently into a ridge detector. One has to squeeze the SPP by an order of magnitude to provide a high mode overlap required for efficient end-fire coupling. This can be achieved by applying a thin SiN x layer on top of the metal ( Fig. 2a ). As shown in Fig. 3c , this enables the excitation of an SPP, which is strongly bound to the interface. In this case, the SPP can be directly coupled into the ridge detector with increased efficiency. We found that the optimal thickness of the SiN x layer in terms of coupling efficiency lies in the same range as required for proper waveguiding (200 nm SiN x ). Figure 3: Excitation and detection of SPPs. ( a ) Without waveguide light couples to free space and partially into the substrate. ( b ) An SPP can be excited on the gold surface, but is weakly bound to the interface. ( c ) The 200-nm-thick SiN x layer on top of the gold surface leads to an increased confinement. Owing to the high confinement, this SPP can be coupled directly to a detector. ( d ) Coupling efficiency from the laser to detector facet over the distance between them, with the simulation as curves and the experiment as points. ( e ) Detector signal into 50 Ω compared with the laser power (front facet) over the laser current density for a distance of 50 μm. The inset shows the time-resolved detector signal. Opt., optical. Full size image We fabricated several devices with different waveguide configurations and distances between the laser and the detector. Figure 3d shows the coupling efficiencies of the fabricated devices compared with the simulations. The coupling efficiency describes the ratio between the power through the detector facet and the power emitted from the laser facet. Without any waveguide, the coupling efficiency drops cubically with increasing distance. With a gold stripe between the laser and the detector, the coupling is improved, but still shows a significant drop at larger waveguide lengths. For the DLSPP waveguide, the coupling efficiency also initially drops because of additional free space coupling, but then approaches a constant slope determined by the waveguide loss. In the simulations, as well as in the experiments, we see a significant dependency on the gap between the ridge facets and the SPP waveguide. For a 50-μm DLSPP waveguide and a gap between the gold surface and the ridge facets of 0.5 and 2.5 μm, we have calculated the coupling efficiency to be 47% and 35%, respectively. All curves show an oscillation because of the presence of longitudinal modes within the SPP waveguide. To minimize coupled cavity effects, the detector facet can be etched with a small lateral angle preventing back reflection into the laser [24] . Alternatively, this effect may be used to force single mode operation. The on-chip detector signal and the laser power versus the laser current density for the device with a distance of 50 μm is plotted in Fig. 3e . The inset shows the time-resolved detector signal of a single pulse at the maximum laser output power. In order to minimize the electric crosstalk between the laser and the detector, we use separated contacts [14] instead of a shared bottom side contact. With a laser power of 200 mW at room temperature (pulse average), we have observed a detector signal of 150 mV into 50 Ω (without amplifier). This corresponds to a coupling efficiency of 35%. The detector voltage signal can be increased to 3 V by terminating it with 1 MΩ rather than 50 Ω. To maintain the bandwidth required to observe 100 ns pulses, the measurement electronics should be placed close or in the direct vicinity of the device. On-chip sensing of chemicals in liquid phase A main challenge in the development of more compact sensor systems is the cost-effective integration of all necessary components while maintaining a good overall performance. However, several advantages compensate for the performance drawbacks that arise from the difficulty to optimize all optical components individually, which underlines the potential of the presented concept. Different to dielectric waveguides, the mode in an SPP waveguide is mainly located outside (96%), providing a high interaction with chemical substances. The end-fire coupling is very efficient compared with conventional optics and enables the use of ridge waveguide detectors. Compared with a discrete QCD, this leads to a signal enhancement because of the increased absorption efficiency. The small size is beneficial for the noise performance of the detector. In order to prove the functionality of our on-chip sensor, we submerged the entire, unpassivated device into a testing fluid consisting of two substances with a low and a high absorption coefficient. For our model experiment, we use ethanol (low absorption at λ =6.5 μm) and distilled water (high absorption at λ =6.5 μm). 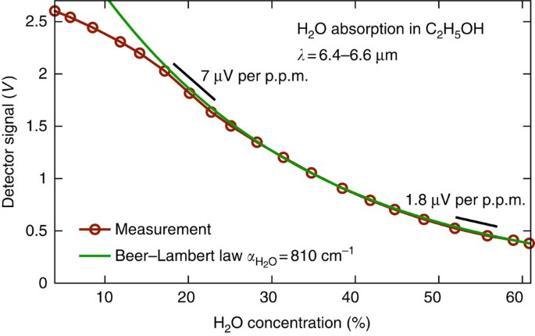Figure 4: On-chip absorption measurement. The entire unpassived sensor device is submerged in a H2O/C2H5OH solution with H2O concentration from 0 to 60%. The detector signal fits to Beer–Lambert law, with a deviation at low concentrations due to detector saturation. Figure 4 shows the detector signal versus the H 2 O concentration of the fluid. A waveguide length of 50 μm is used to cover a high dynamic range of concentrations from 0 to 60% with a slope of 1.8–7 μV per p.p.m., which can be easily analysed with state-of-the-art electronics. Although longer waveguides are preferable to increase the sensitivity for low concentrations, short interaction length are beneficial if the background absorption is high, for example, water containing liquids or high concentrations of the chemicals. Figure 4: On-chip absorption measurement. The entire unpassived sensor device is submerged in a H 2 O/C 2 H 5 OH solution with H 2 O concentration from 0 to 60%. The detector signal fits to Beer–Lambert law, with a deviation at low concentrations due to detector saturation. Full size image The absorption coefficient of H 2 O obtained by fitting to Beer–Lambert’s law agrees well with literature data [25] . At small concentrations, the slope is slightly smaller owing to detector saturation. Detector saturation occurs in voltage mode, when a voltage amplifier with a high input impedance (1 MΩ) is used ( Supplementary Fig. 1 ). In this case, the photocurrent leads to a voltage drop V QCD ≈ R QCD I ph across the heterostructure, which significantly alters the bandstructure. As the detector was designed for operation near zero bias, the high reverse bias affects the absorption peak position, the extraction efficiency and the differential resistance. The laser power can be reduced that would lead to a higher resolution at low concentrations, but a lower resolution at high concentrations. In current mode, the QCD is terminated with a small resistance that decreases the voltage drop across the heterostructure and guaranties the operating condition near zero bias. In this case, we have not observed any detector saturation that allows a better resolution at low concentrations. When the entire device is submerged into the fluid, the refractive index of the carrier fluid alters the reflectivity of the facets and the waveguide properties, but all components remain functional. The confinement of the DLSPP is only slightly modified. For sensing operation, the change of the reflectivity because of the analyte in the carrier fluid can be neglected compared with the more pronounced absorption features. A small remaining effect may be corrected using a calibration curve. Although not necessarily required, a high-reflectivity coating was applied during the contact fabrication to minimize the impact of the fluid onto the back facet. Owing to the typical relatively low conductivity of fluids, an insulation is not necessarily required. To insulate the device or to improve its chemical stability over the solvent or analyte, the device can be passivated with a thin dielectric layer, for example, SiO 2 or CaF 2 . Regular purging, for example, with acetone or isopropyl alcohol, can be used to prevent false positives due to waveguide or detector poisoning. We tested a 150-nm-thick SiO 2 passivation layer covering the entire wire-bonded device and reinforced the bond wires with polyamide, without a significant performance reduction. Certainly, the passivation layer should have a small refractive index to maintain the lateral index contrast of the SPP waveguide ( ) [26] and has to be considered in the waveguide design. Another possible passivation material would be CaF 2 with a refractive index of , which is known to be chemically stable. Alternatively, the sensor can be combined with microfluidics, fabricating a fluidic channel on top of the waveguide. A common way to express the resolution of chemical sensors is the limit of detection that denotes the smallest detectable concentration Δ c . Without any pulse-to-pulse normalization, the limit of detection with a 3 σ criteria can be calculated to be , with σ P / P 0 =2% pulse-to-pulse fluctuation, α is the absorption coefficient of the analyte L eff =0.96 × 50 μm is the effective interaction length and N is the number of averaged pulses. In the prototype test setup, we averaged over N =512 pulses, which results in a limit of detection of Δ c =0.06% over the entire range from 0 to 60% and beyond. The accuracy can be further increased by even longer averaging. At a certain point, other effects limit the performance, such as drift due to temperature fluctuations of the device and the measurement electronics. As in every laser-based optical absorption measurement system, a fluctuation of the laser and detector temperature results in a change of the detected signal. Around room temperature, the entire device shows a sensitivity to temperature fluctuations of σ V / V 0 =2.45% per °C. The device temperature is thermoelectrically controlled to 22±0.01 °C that results in a limit of detection of Δ c =3 σ V ( V 0 α L eff ) −1 =0.02%. As a common solution in chemical sensing, pulse-to-pulse intensity fluctuations as well as temperature-induced fluctuations can be accounted for by using a second reference detector [27] that can be integrated at the back facet of the laser. Owing to the operation at zero bias, the noise of QCDs is commonly dominated by thermal noise [15] . With the high device resistance of R 0 =1.7 kΩ, the thermal noise can be calculated to be . Rather unexpected, this is not the limiting noise mechanism. It is the shot noise generated by the signal itself that limits the noise performance. Owing to the discrete nature of electrons, the signal current is overlayed by the noise current . The 3 σ limit of detection for 100 ns pulses is , where R is the detector responsivity. Owing to the high detector signal, amplifier noise is not a limiting factor, although drift of the measurement electronic might be a limiting mechanism. The presented model experiment clearly demonstrates the functionality and competitive performance of the presented device concept. We achieved a resolution of Δ c =0.06% over a huge dynamic range from 0 to 60%, which can be further improved with a second detector at the back facet to correct pulse-to-pulse intensity and thermally induced fluctuations. It must be pointed out, in this experiment, that high accuracy can only be achieved if the mixture is known to contain only ethanol and water. In cases, where the constituents of the analyte are known but need to be quantified, a properly designed QCL-SPP-QCD structure can serve as a simple, cost-effective sensor. Whenever selectivity or identification of substances is required, this concept can be easily extended through multi-wavelength configurations. This can be achieved by designing the gain and detection region to cover the relevant wavelength range. Since the bi-functional active region is based on a bound-to-continuum transition, the laser provides a broad spectral gain of ~\n100 cm −1 , which may be further increased with particular design techniques [28] , [29] . To address the specific molecular resonances, two or more laser waveguide detector units on the same chip with different distributed feedback gratings on the lasers can be fabricated [30] , circumventing beam combining issues. A continuous spectral coverage can be obtained by intrapulse wavelength tuning due to device heating [31] . Although not required for fluidic sensing because of the relatively broad absorption features, the fast response of the on-chip detector is beneficial to achieve a high spectral resolution. We demonstrated a mid-infrared on-chip sensor based on absorption spectroscopy. Our monolithic device comprises a laser, an SPP waveguide as well as a detector integrated on a single chip. For the laser and the detector, we use a bi-functional QCLD. This active region can be used either as a laser or a detector depending on the applied bias. The laser light is coupled through an SPP waveguide, acting as interaction zone, to the detector. Owing to the evanescent nature of SPPs, 96% of the mode stays outside and interacts with the chemicals. The waveguide is fabricated with a thin dielectric stripe (200 nm) on top of an unpatterned gold surface, thereby solving two major issues. First, the weakly confined mid-infrared SPPs are squeezed, enabling the propagation of strongly bound SPPs and their direct coupling from and to ridge waveguides. Second, by eliminating the metal edges in the waveguide, the propagation length of narrow SPP waveguides (15 μm) is increased by one order of magnitude. The fabricated devices with 50 and 100 μm waveguide lengths show coupling efficiencies (from the laser to the detector) of 30–50%. At room temperature, the laser has a peak output power of 200 mW and the on-chip detector has an internal quantum efficiency of 33%. Owing to direct coupling from the waveguide and the optimized quantum design, the on-chip detector provides a better performance than discrete QCDs. In order to demonstrate the functionality of the on-chip sensor, we submerged the device into a H 2 O/C 2 H 5 OH solution. With a waveguide length of 50 μm, the device covers a high dynamic range of concentrations (0–60%). Without any compensation for pulse-to-pulse intensity fluctuations, we achieve a sensing resolution of 0.06%. This clearly demonstrates that monolithic integration is not necessarily connected with large performance limitations. Furthermore, our approach allows a straightforward and cost-saving fabrication, as no subwavelength patterning or special hybrid integration approach is necessary. The presented device can thus be used as an extremely compact, cost-efficient device for high dynamic range sensing with capabilities to reach p.p.m. accuracy. Simulation The optical simulations were carried out with the commercial simulation tool COMSOL Multiphysics ( www.comsol.com ). For gold and SiN x , we used a refractive index at λ =6.5 μm of n =3.3–46.7 i and n =1.85–0.003 i extrapolated from literature [21] , [32] , respectively. The optical properties of the semiconductor materials were calculated using the Drude model. The evanescent decay length was extracted from the numerical simulations via fitting to an exponentially decaying function. The propagation length in Fig. 2d was extracted from the imaginary part of the modal index, as shown in Fig. 2b,c . The absorption coefficient α and the extraction efficiency p e of the QCD were calculated using a single-particle Monte–Carlo transport simulator for quantum cascade devices [33] , resulting α =200 cm −1 and p e =43% at room temperature, respectively. With COMSOL Multiphysics, we then obtained an absorption efficiency η for the 200-μm long ridge detector of ~\nη=77% (absorbed power, which passed the detector facet). Fabrication A bi-functional QCLD active region with a InAlAs top cladding layer was grown on a n-doped InP substrate by solid source molecular beam epitaxy. The heterostructure based on the bound-to-continuum design, consists of 37 cascades of In 0.52 Al 0.48 As/In 0.53 Ga 0.47 As lattice matched to InP. The layer sequence, starting from the injector barrier, is as follows: 4.3 /1.3/ 1.5 /5.2/ 2.5 /4.2/ 2.6 /3.5/ 2.8 /3.1/ 3.0 /2.8/ 2.7 /2.7/ 2.7 /2.6/ 2.7 /2.4/ 2.7 /2.2/ 2.7 /1.9/ 3.4 /1.9/ 2.7 /1.7 nm. The barrier layers are in bold and the underlined layers are n-doped with Si 2 × 10 17 cm −3 . The 15-μm-wide laser and detector ridges, as well as a gap between them were dry etched by reactive ion etching in SiCl 4 atmosphere at 220 °C, whereby SiN x was used as a hard mask. The distance between the laser and the detector is 5, 50 and 100 μm long. The depth of the ridge is 6 μm, as it was etched through the active zone to the substrate. The lasers and detectors were isolated from each other by evaporating 500 nm SiN x , whereby electrical contacts area and ridge facets towards the waveguide remains uncovered. Instead of a bottom side substrate contact, we used adjacent contacts in the trenches beside the ridges in order to minimize electric crosstalk via a shared series resistance [14] . Ohmic contacts were formed by e-beam evaporation of Ge/Au/Ni/Au (15/30/14/100 nm). Afterwards, layers of titanium and gold, 10 and 400 nm thick, respectively, were sputtered to form the SPP waveguides, the extended contacts and a high-reflectivity coating on the back facets. It improves the adhesion to SiN x passivation layer and provides better coverage of the ridge side walls due to resputtering. Finally, 200 nm of SiN x was deposited and etched as a stripe to from the DLSPP waveguides. To investigate the impact of the gap between the ridge facets and the SPP waveguides, we fabricated different gaps of 0.5 and 2.5 μm. The laser and detector ridges are 2.5 mm and 200 μm long, respectively. For Fig. 3d,e , the back facet of the laser was cleaved to enable a measurement of the laser emission with an external detector, resulting in a ridge length of 2.4 mm. Measurements All experimental results were performed at room temperature (22 °C) controlled by a Peltier element. The lasers were operated in pulsed mode, with a pulse length of 100 ns and a repetition rate of 5 kHz. The optical power of the laser was measured with a calibrated deuterated triglycine sulfate (DTGS) detector within a Bruker FTIR ( Fig. 3d,e ). Voltage and current measurements were performed using a Tektronix TDS 3032B digital oscilloscope and a shunt resistor. The laser was connected with a series resistance of 47 Ω that, together with the QCL, matches the coaxial cable impedance. The second direct port was used to measure the detector voltage and was terminated with a 50 Ω ( Fig. 3d,e ) or 1 MΩ ( Fig. 4 ) resistance. How to cite this article: Schwarz, B. et al. Monolithically integrated mid-infrared lab-on-a-chip using plasmonics and quantum cascade structures. Nat. Commun. 5:4085 doi: 10.1038/ncomms5085 (2014).